SOX2 is a cancer-specific regulator of tumour initiating potential in cutaneous squamous cell carcinoma Although the principles that balance stem cell self-renewal and differentiation in normal tissue homeostasis are beginning to emerge, it is still unclear whether cancer cells with tumour initiating potential are similarly governed, or whether they have acquired distinct mechanisms to sustain self-renewal and long-term tumour growth. Here we show that the transcription factor Sox2, which is not expressed in normal skin epithelium and is dispensable for epidermal homeostasis, marks tumour initiating cells (TICs) in cutaneous squamous cell carcinomas (SCCs). We demonstrate that Sox2 is required for SCC growth in mouse and human, where it enhances Nrp1/Vegf signalling to promote the expansion of TICs along the tumour–stroma interface. Our findings suggest that distinct transcriptional programmes govern self-renewal and long-term growth of TICs and normal skin epithelial stem and progenitor cells. These programmes present promising diagnostic markers and targets for cancer-specific therapies. Identification of self-renewing cancer stem cells (CSCs), uniquely capable of sustaining long-term growth of hierarchically organized cancers [1] , implies that cancer therapies that target and destroy CSCs may cure rather than just temporarily contain the disease [2] . The development of such CSC-specific therapies, however, depends on the identification of CSCs and the molecular mechanisms that are essential for their viability, self-renewal and long-term tumour initiating potential, while they are at the same time dispensable for normal tissue stem cell functions. Skin epithelium and cutaneous squamous cell carcinoma (SCC) present powerful model systems in which to investigate whether stemness is governed by the same or distinct molecular mechanisms in homeostasis and carcinogenesis. In the skin epithelium, a number of stem and progenitor cell populations have been identified [3] , [4] , [5] , [6] , [7] , [8] . Most prominent are hair follicle stem cells (HFSCs) that are located in the, permanent part of the hair follicle known as bulge. HFSCs have first been defined based on their slow-cycling behaviour [9] and elevated colony-forming potential [10] , which enabled the identification of transcriptional [11] , [12] and epigenetic [13] signatures that distinguish HFSCs from other skin epithelial cell types. HFSCs have been isolated based on their expression of the cell surface proteins α6 and β1 integrin, as well as CD34, cultured on 3T3 feeder layers long term and differentiated into all skin epithelial cell lineages after transplantation onto Nude mice [14] . These properties defined HFSCs as stem cells and distinguished them from other skin epithelial cell lineages with limited proliferative potential [15] . Similarly, cutaneous SCC, a hierarchically organized skin cancer that can originate from HFSCs as well as other skin epithelial cells [16] , [17] , [18] , is sustained by cancer cells with tumour initiating potential, which self-renew and also differentiate into tumour cells without the ability to form tumours after transplantation [19] . Tumour initiating cells (TICs) in murine cutaneous SCC have been identified at the tumour–stroma interface where they express high levels of α6 and β1 integrin, as well as CD34 (refs 20 , 21 ). These cells are able to initiate and propagate SCCs that resemble the phenotypic heterogeneity of their parent in serial transplantation experiments. Differential gene expression analyses defined a characteristic molecular signature that distinguishes TICs in SCCs from normal skin epithelial stem and progenitor cells [20] . Intriguingly, essential HFSC regulators, including Lhx2 (LIM homeobox 2), which maintains HFSC function [22] , Tbx1 (T-box protein 1), which governs their self-renewal [23] , and Nfatc1 (nuclear factor of activated T cells 1), which restricts their activation [24] and functions as a tumour suppressor gene [25] , are strongly repressed or undetectable in TICs of murine SCCs [20] ( Fig. 1a ). This observation suggested the hypothesis that self-renewal and long-term growth of SCC initiating tumour cells may be governed by molecular mechanisms that are distinct from normal skin epithelial stem and progenitor cells from which the tumours originated. 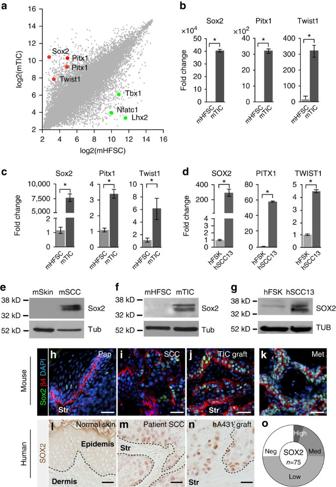Figure 1: SOX2 expression distinguishes TICs from normal skin epithelial cells. (a) Scatter plot illustrating gene expression values of 45,101 transcripts in TICs of murine (m) cutaneous SCC compared with HFSCs. Red and green dots indicate highly enriched transcription factors in mTICs and mHFSCs, respectively. (b) qRT–PCR analyses of Sox2, Pitx1 and Twist1 on RNA from freshly sorted mTICs and mHFSCs. (c) qRT–PCR analysis of Sox2, Pitx1 and Twist1 on RNA from cultured mTICs and mHFSCs. (d) qRT–PCR analysis of SOX2, PITX1 and TWIST1 on RNA from human foreskin (FSK) and SCC13 cultures. (b–d) Data are represented as mean with error bars indicating ±s.d. (n=3, *P<0.05, Student’st-test). (e–g) Western blot analyses of Sox2 on total protein extracts from mSkin and mSCC (e); cultured mHFSCs and mTIC (f); and human foreskin keratinocyte (FSK) and SCC13 cultures (g). β-Tubulin (Tub) was used as loading control. (h–k) Immunofluorescence microscopy of Sox2 (green) on benign mouse papillomas (h, Pap), primary mouse SCCs (i, SCC), orthotopic TIC transplants (j, TIC graft) and spontaneous lung metastases (k, Met). β4 integrin (red) demarcates the boundary between tumour epithelial cells and underlying stroma (Str). DAPI (blue) labels nuclear chromatin. (l–n) Immunohistochemistry of SOX2 on normal human skin (l), primary human patient SCC (m) and A431 xenograft (n). (o) Donut chart summarizing SOX2 expression analysis on human cutaneous SCC tissue microarray. Nuclear SOX2 staining was detected in 75% of SCCs (56/75) with variable staining intensity (5% strong, 20% medium, 49% weak). (h–n) Scale bars, 50 μm. Figure 1: SOX2 expression distinguishes TICs from normal skin epithelial cells. ( a ) Scatter plot illustrating gene expression values of 45,101 transcripts in TICs of murine (m) cutaneous SCC compared with HFSCs. Red and green dots indicate highly enriched transcription factors in mTICs and mHFSCs, respectively. ( b ) qRT–PCR analyses of Sox2, Pitx1 and Twist1 on RNA from freshly sorted mTICs and mHFSCs. ( c ) qRT–PCR analysis of Sox2, Pitx1 and Twist1 on RNA from cultured mTICs and mHFSCs. ( d ) qRT–PCR analysis of SOX2, PITX1 and TWIST1 on RNA from human foreskin (FSK) and SCC13 cultures. ( b – d ) Data are represented as mean with error bars indicating ±s.d. ( n =3, * P <0.05, Student’s t -test). ( e – g ) Western blot analyses of Sox2 on total protein extracts from mSkin and mSCC ( e ); cultured mHFSCs and mTIC ( f ); and human foreskin keratinocyte (FSK) and SCC13 cultures ( g ). β-Tubulin (Tub) was used as loading control. ( h – k ) Immunofluorescence microscopy of Sox2 (green) on benign mouse papillomas ( h , Pap), primary mouse SCCs ( i , SCC), orthotopic TIC transplants ( j , TIC graft) and spontaneous lung metastases ( k , Met). β4 integrin (red) demarcates the boundary between tumour epithelial cells and underlying stroma (Str). DAPI (blue) labels nuclear chromatin. ( l – n ) Immunohistochemistry of SOX2 on normal human skin ( l ), primary human patient SCC ( m ) and A431 xenograft ( n ). ( o ) Donut chart summarizing SOX2 expression analysis on human cutaneous SCC tissue microarray. Nuclear SOX2 staining was detected in 75% of SCCs (56/75) with variable staining intensity (5% strong, 20% medium, 49% weak). ( h – n ) Scale bars, 50 μm. Full size image Here we identify three transcription factors, including Sox2 (SRY (sex determining region Y) box 2) Pitx1 (paired like homeodomain transcription factor 1) and Twist1 (twist basic helix-loop-helix transcription factor 1), which are expressed in mouse and human SCCs, while they are not detectable in normal skin epithelial cells. We find Sox2-expressing SCC cells within the α6 and β1 integrin-expressing cell population lining the tumour–stroma interface. Sox2 expression is critical for tumour initiation and growth, as it promotes the expansion of tumour initiating SCC cells along the tumour–stroma interface. Sox2 expression identifies TICs of cutaneous SCCs To discover molecular markers unique to TICs, we directly compared global gene expression profiles of mouse epidermal SCC TICs with HFSCs ( Fig. 1a ) and epidermal progenitor cells (Epi, Supplementary Fig. 1a ) [20] . Among the molecules that are consistently expressed in all TIC populations, with expression tightly repressed in normal skin epithelial stem and progenitor cells, as well as in their differentiating progeny, are three transcription factors: Sox2, Pitx1 and Twist1 ( Fig. 1a and Supplementary Fig. 1 ). In contrast, the HFSC regulators Lhx2, Tbx1 and Nfatc1 are strongly repressed or undetectable in SCC TICs. The differential expression of these identified molecular markers was further confirmed by quantitative reverse-transcription PCR (qRT–PCR) analyses on freshly isolated TICs and HFSCs ( Fig. 1b and Supplementary Fig. 2 ). Next, we established primary cultures from TICs and HFSCs, which are able to proliferate over many passages in vitro reflecting their long-term self-renewing potential. We then evaluated the relative expression of our candidate genes in both cultures by qRT–PCR analyses. Expression of Sox2, Pitx1 and Twist1 was significantly elevated in cultured TICs compared with primary keratinocyte cultures established from HFSCs ( Fig. 1c ), while the HFSC self-renewal gene Tbx1 (ref. 23 ), and the embryonic stem cell (ESC) self-renewal genes and Sox2 partners Oct4 and Nanog [26] , remained repressed in cultured TICs ( Supplementary Fig. 3 ). We surmised that if Sox2, Pitx1 and Twist1 are indeed required for the self-renewing potential of TICs in SCC, then they should also be expressed in tumour initiating human SCC cell lines [27] , [28] . Indeed, qRT–PCR analyses confirmed the elevated expression of SOX2, PITX1 and TWIST1 in human SCC lines when compared with normal human keratinocyte cultures ( Fig. 1d and Supplementary Fig. 4a ). Furthermore, western blotting analyses for Sox2 also showed significant enrichment in SCC compared to whole skin protein extracts, as well as lysates of mouse and human SCC cultures when compared with normal keratinocyte cultures, confirming our results at the protein level ( Fig. 1e–g and Supplementary Fig. 4b ). SOX2 expressing SCC cells reside at the tumour–stroma interface To determine the location of Sox2-expressing cells in mouse and human tumour specimens, we analysed their distribution by immunofluorescence microscopy and immunohistochemistry. Confirming our Sox2 expression analyses in sorted normal and tumour tissue cell fractions, Sox2 was not found by immunofluorescence in normal skin epithelium [29] , [30] but it was readily detected in murine tumours ( Fig. 1h–k ). In benign papillomas, Sox2 was expressed in a few undifferentiated tumour cells that reside at the tumour–stroma interface, but it was more readily observed within their differentiating progeny ( Fig. 1h ). In primary SCCs, however, Sox2 expression was consistently detected (20/20) in nuclei of undifferentiated SCC cells, which clustered in areas at the tumour–stroma interface, where they express high levels of the basal cell markers α6 and β1 integrin ( Fig. 1i ). Intriguingly, the focal localization of nuclear Sox2-expressing SCC cells was expanded to include the majority of undifferentiated tumour cells in secondary SCCs, which developed after transplantation of α6 and β1 integrin-expressing SCC cells onto Nude hosts ( Fig. 1j ). Likewise, nuclear Sox2 expression was also detected in the majority of undifferentiated keratin 14-positive cells in spontaneous lung metastases (5/5), which formed in <5% of our 7,12-dimethylbenz(a)anthracene (DMBA)-treated mice ( Fig. 1k and Supplementary Fig. 5 ). A similar differential expression pattern was also observed in human skin and primary human SCCs ( Fig. 1l–o and Supplementary Fig. 6 ). SOX2 expression was not detectable in normal human skin epithelium ( Fig. 1l ) but it was frequently found in clusters of undifferentiated tumour cells residing at the tumour–stroma interface of patient-derived SCCs and in tumours grown after xenotransplantation of human SCC cell lines onto Nude mice ( Fig.1m,n ). Indeed, nuclear Sox2 expression was prevalent in 75% of patient-derived SCCs, but it varied in expression levels and abundance between specimens ( Fig. 1o and Supplementary Fig. 6 ). Together, the differential and prevalent expression of Sox2 in mouse and human cutaneous SCCs and its enrichment in TICs suggests Sox2 as a novel molecular marker that distinguishes TICs from normal skin epithelial stem and progenitor cells. Epigenetic changes enable de novo Sox2 expression in SCC A priori , this de novo expression of Sox2 in cutaneous SCCs could result from genetic as well as epigenetic changes. To test whether elevated Sox2 expression in SCC TICs compared with normal skin epithelial stem and progenitor cells is due to genomic amplification as recently reported for human oesophageal and lung SCCs [31] , [32] , we determined the copy number variation by TaqMan qRT–PCR assays. Our measurements revealed no genomic amplification of the Sox2 locus in mouse and human cutaneous SCC cultures ( Supplementary Fig. 7a ). Indeed, Sox2 is expressed in normal oesophageal stem and progenitor cells as well as in lung epithelial cells during homeostasis [29] , while histone H3 lysine 27 trimethylation (H3K27me3) of the Sox2 promoter indicates transcriptional repression in skin epithelial stem and progenitor cells [13] , [33] . To test whether the de novo expression of Sox2 in cutaneous SCC TICs is due to a loss in H3K27me3, we determined whether the Sox2 promoter carries this repressive chromatin mark by chromatin immunoprecipitation (ChIP)–PCR. Our analysis revealed that the repressive H3K27me3 mark was significantly reduced in TIC compared with HFSC-derived keratinocyte cultures consistent with the de novo expression of Sox2 ( Supplementary Fig. 7b ). Intriguingly, the reduction in H3K27me3 repression appears to be locus specific rather than genome wide, because H3K27me3 levels were elevated at other gene promoters and on total protein extracts of SCC TIC compared with HFSC-derived keratinocyte cultures ( Supplementary Fig. 7b,c ). Furthermore, Polycomb Repressive Complex components were expressed in both TICs of cutaneous SCCs and normal skin epithelial stem and progenitor cells ( Supplementary Fig 7d ). SOX2 promotes SCC initiation and growth To test whether SOX2 expression is required for SCC growth, we infected human SCC lines and primary murine TICs with lentivirus expressing histone 2B-red fluorescent protein (H2B-RFP) along with a short hairpin RNA (shRNA) that efficiently reduced SOX2 mRNA and protein levels ( Supplementary Fig. 8a–c ). Lentivirus expressing scrambled (SCR) shRNA along with histone 2B-green fluorescent protein (H2B-GFP) was used as control [34] . Control (shSCR) and SOX2 knockdown (shSOX2) cells were transplanted onto Nude recipient mice, where control-infected tumours grew rapidly and at a similar rate to uninfected SCCs, while SOX2 depletion resulted in delayed and significantly reduced SCC growth ( Fig. 2a and Supplementary Fig. 8d ). Intriguingly, only (8/16) tumours initiated following transplantation and 2 of these tumours regressed after initial signs of tumour growth. 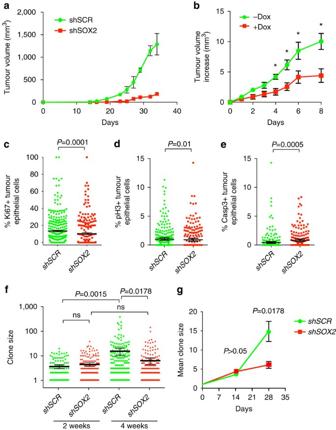Figure 2: SOX2 is required for cutaneous SCC initiation and growth. (a) Tumour growth curves of human SCCs infected with lentivirus expressing shRNA against SOX2 along with nuclear red fluorescent protein (H2B-RFP; shSOX2) or SCR control shRNA along with nuclear green fluorescent protein (H2B-GFP; shSCR) followed by transplantation onto Nude recipient mice. Data are represented as mean with error bars indicating ±s.e.m. (n=6, *P<0.05, Student’st-test). (b) Doxycycline-inducible knockdown of SOX2 in established human SCC xenografts. Data are represented as mean with error bars indicating ±s.e.m. (n=10, *P<0.05, Student’st-test). (c–e) Quantitative analysis of proliferative Ki67 (c), mitotic phospho-Histone H3-Ser10 (pH3). (d) and apoptotic activated Caspase-3 (Casp3)- (e) positive cells in shSOX2;H2B-RFP or shSCR;H2B-GFP-transduced A431 xenografts. Scatter plots illustrate the percentage of infected parenchymal cells that are positive for the respective marker inn>200 microscopic fields. Horizontal bars indicate mean ±95% confidence interval (CI). (*P<0.05 Mann–Whitney non-parametrict-test). (f,g) Analysis of clonal growth competition assay at 2 and 4 weeks after intradermal transplantation when 1–2% of A431 cells have been transduced with shSOX2;H2B-RFP and shSCR;H2B-GFP (n=6). (f) Scatter plots illustrate clone size distributions. Horizontal lines represent mean with error bars indicating ±95% CI. (g) Line graphs showing average clone size as a function of time (±s.e.m). (f,g)P-values were obtained by Mann–Whitney non-parametrict-tests. Figure 2: SOX2 is required for cutaneous SCC initiation and growth. ( a ) Tumour growth curves of human SCCs infected with lentivirus expressing shRNA against SOX2 along with nuclear red fluorescent protein (H2B-RFP; shSOX2) or SCR control shRNA along with nuclear green fluorescent protein (H2B-GFP; shSCR) followed by transplantation onto Nude recipient mice. Data are represented as mean with error bars indicating ±s.e.m. ( n =6, * P <0.05, Student’s t -test). ( b ) Doxycycline-inducible knockdown of SOX2 in established human SCC xenografts. Data are represented as mean with error bars indicating ±s.e.m. ( n =10, * P <0.05, Student’s t -test). ( c – e ) Quantitative analysis of proliferative Ki67 ( c ), mitotic phospho-Histone H3-Ser10 (pH3). ( d ) and apoptotic activated Caspase-3 (Casp3)- ( e ) positive cells in shSOX2;H2B-RFP or shSCR;H2B-GFP-transduced A431 xenografts. Scatter plots illustrate the percentage of infected parenchymal cells that are positive for the respective marker in n >200 microscopic fields. Horizontal bars indicate mean ±95% confidence interval (CI). (* P <0.05 Mann–Whitney non-parametric t -test). ( f , g ) Analysis of clonal growth competition assay at 2 and 4 weeks after intradermal transplantation when 1–2% of A431 cells have been transduced with shSOX2;H2B-RFP and shSCR;H2B-GFP ( n =6). ( f ) Scatter plots illustrate clone size distributions. Horizontal lines represent mean with error bars indicating ±95% CI. ( g ) Line graphs showing average clone size as a function of time (±s.e.m). ( f , g ) P -values were obtained by Mann–Whitney non-parametric t -tests. Full size image The severe reduction in tumour growth following SOX2 depletion suggested a critical role for SOX2 in tumour initiation and/or maintenance. To address whether SOX2 function is still required once SCCs are established, we transplanted human and mouse TICs infected with a lentivirus encoding a doxycycline-regulated shSOX2 onto Nude mice. Induction of shSOX2 in fully formed tumours resulted in a significant reduction in growth of both human ( Fig. 2b ) and murine ( Supplementary Fig. 8e ) SCC grafts. To investigate the cellular defects responsible for the reduced tumour growth, we measured the relative rates of proliferation and apoptosis in control and SOX2-depleted SCC grafts. SCC sections were stained with the proliferation markers Ki67 ( Fig. 2c ) and phospho-histone H3-Ser10 ( Fig.2d ), as well as active caspase 3 ( Fig. 2e ), to detect apoptotic cells within the H2B-GFP- or H2B-RFP-labelled tumour epithelium. shSOX2 knockdown SCCs showed a small but significant decrease in proliferative tumour epithelial cells and a significant increase in apoptotic figures. We surmised that SOX2 could promote SCC growth by cell intrinsic as well as extrinsic mechanisms. To test this hypothesis, we performed clonal competition and lineage trace studies in our human ( Fig. 2f,g ) and mouse ( Supplementary Fig. 8f,g ) SCC transplantation models. We produced a mixture of control (shSCR-GFP) and knockdown (shSOX2-RFP) lentivirus, and infected TICs at clonal density, so that only a small percentage of cells were transduced. To ensure that equal green fluorescent protein/red fluorescent protein (GFP/RFP) numbers of sparsely transduced cells were transplanted, we measured the transduction efficiency by flow cytometry before their injection into Nude recipient mice. We then allowed the transplants to develop into tumours, which we processed to directly compare the growth characteristics of SOX2-positive and SOX2-negative clones within the same tumour. Interestingly, clone size measurements revealed no significant differences between control and SOX2 knockdown clones within the first 2 weeks of tumour growth ( Fig. 2f,g and Supplementary Fig. 8f,g ). However, 4 weeks after transplantation, SOX2-depleted clones were significantly smaller when compared with control ( P <0.0001; Fig. 2f,g and Supplementary Fig. 8f,g ). In addition to quantitative immunofluorescence microscopy of transduced SCC clones, we performed a series of flow cytometric analyses, measuring the ratios of Sox2-depleted and control cells in SCCs over time. These experiments confirmed that although the ratio of Sox2-negative/positive cells remains unchanged during the initial growth period, Sox2 knockdown cells are eventually outcompeted by Sox2-positive cells ( Supplementary Fig. 8h ). Similar results were obtained in clonal competition experiments in culture ( Supplementary Fig. 8i ). The severe reduction in SCC growth following Sox2 knockdown indicated an essential function in SCC initiation and maintenance. To test whether ectopic Sox2 expression is sufficient to initiate and drive SCC growth, we infected primary HFSC-derived keratinocyte cultures with lentivirus expressing Sox2 under the ubiquitous PGK promoter followed by their transplantation into Nude mice. Keratinocytes infected with LZRS-Ras G12V were used as a positive control. In contrast to LZRS-Ras G12V -infected HFSCs, which formed tumours efficiently following transplantation into Nude mice [35] , ectopic expression of Sox2 alone was not sufficient to initiate skin carcinogenesis ( Supplementary Fig. 8j ). Together, our data indicate that Sox2 is critical for SCC growth, but insufficient to initiate skin carcinogenesis. To better understand how Sox2 promotes SCC growth at the molecular level, we compared the gene expression signature that distinguishes TICs from normal skin epithelial stem and progenitor cells [20] ( Fig. 1a ) with direct Sox2 target genes in ESCs [36] . This analysis identified 466 putative Sox2 targets ( Fig. 3a and Supplementary Data 1 ), including the transcription factor Pitx1 and the pro-angiogenic factors neuropilin (Nrp1, Nrp2) [37] , secreted phosphoprotein 1 (Spp1) [38] , phosphatidylinositol transfer protein cytoplasmic 1 (Pitpnc1) [39] and insulin growth factor 2 binding protein 2 (Igf2bp2), as genes with the highest differential expression in SCC TICs ( Fig. 3b,c ). To establish whether their expression is dependent on Sox2 function, we first verified their elevated expression in TICs compared with HFSCs by qRT–PCR ( Fig. 3d ). We then measured their expression in Sox2 knockdown TICs compared with Scr controls. Indeed, all of our candidate genes were detected at significantly lower expression levels when Sox2 was depleted—consistent with a function for Sox2 in regulating their expression in TICs ( Fig. 3e ). In addition, we performed ChIP–PCR experiments and demonstrated a significant enrichment of Sox2 protein at the enhancer sequences of these genes ( Fig. 3f ). Notably, Sox2 also promoted the expression of vascular endothelial growth factor A (Vegfa) and the epidermal growth factor receptor ligands Epiregulin (Ereg) and tumour growth factor-α (Tgfa) ( Fig. 3g,h ), which are contained in our list of signature genes that are expressed in TICs but not in HFSCs ( Supplementary Fig. 1c ). 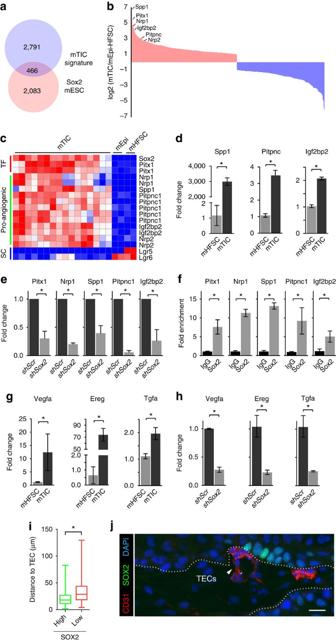Figure 3: Sox2 promotes the expression of pro-angiogenic factors in TICs. (a) Venn diagram depicting overlap of 466 genes between the mouse TIC signature and a list of direct Sox2 targets in mouse ES cells. (b) Histogram illustrating the relative enrichment of 466 putative Sox2 target genes in mouse TICs compared with skin epithelial stem and progenitor cells. Two hundred and fifty four genes are >2-fold upregulated (red) and 212 genes are >2-fold downregulated (blue). Pro-angiogenic molecules and Pitx1 are among the highest differentially expressed genes. (c) Heat map exemplifying elevated expression of Pitx1 and pro-angiogenic factors, and the suppression of HFSC markers in TICs. (d) qRT–PCR analysis of Spp1, Pitpnc and Igf2bp2 on TIC and HFSC cultures. (e) qRT–PCR analysis of Pitx1 and pro-angiogenic factors on mTIC cultures transduced with shScr or shSox2. (f) qRT–PCR analyses on chromatin samples from cultured mTICs after immunoprecipitation with anti-Sox2 and IgG control antibodies. (g) qRT–PCR analysis of EGF and VEGF signalling pathway components on primary mTICs and mHFSC cultures. (h) qRT–PCR analysis of EGF and VEGF signalling pathway components on mTIC cultures transduced with shScr or shSox2. (d–h) Bar graphs showing mean with error bars indicating ±s.d. (n=3, *P<0.05 Student’st-test). (i) Box and whisker plots describing measurements of the closest distance between TICs, expressing high or low levels of SOX2, and tumour endothelial cells (TECs). Bar indicates median, box indicates 25 and 75 percentile, and whiskers indicate minimum and maximum measurements. (j) Representative image showing high-level SOX2-positive cells (green), TECs (CD31, red) and nuclear chromatin (DAPI, blue). White dotted line indicates tumour–stroma interface. Scale bar, 20 μm. Figure 3: Sox2 promotes the expression of pro-angiogenic factors in TICs. ( a ) Venn diagram depicting overlap of 466 genes between the mouse TIC signature and a list of direct Sox2 targets in mouse ES cells. ( b ) Histogram illustrating the relative enrichment of 466 putative Sox2 target genes in mouse TICs compared with skin epithelial stem and progenitor cells. Two hundred and fifty four genes are >2-fold upregulated (red) and 212 genes are >2-fold downregulated (blue). Pro-angiogenic molecules and Pitx1 are among the highest differentially expressed genes. ( c ) Heat map exemplifying elevated expression of Pitx1 and pro-angiogenic factors, and the suppression of HFSC markers in TICs. ( d ) qRT–PCR analysis of Spp1, Pitpnc and Igf2bp2 on TIC and HFSC cultures. ( e ) qRT–PCR analysis of Pitx1 and pro-angiogenic factors on mTIC cultures transduced with shScr or shSox2. ( f ) qRT–PCR analyses on chromatin samples from cultured mTICs after immunoprecipitation with anti-Sox2 and IgG control antibodies. ( g ) qRT–PCR analysis of EGF and VEGF signalling pathway components on primary mTICs and mHFSC cultures. ( h ) qRT–PCR analysis of EGF and VEGF signalling pathway components on mTIC cultures transduced with shScr or shSox2. ( d – h ) Bar graphs showing mean with error bars indicating ±s.d. ( n =3, * P <0.05 Student’s t -test). ( i ) Box and whisker plots describing measurements of the closest distance between TICs, expressing high or low levels of SOX2, and tumour endothelial cells (TECs). Bar indicates median, box indicates 25 and 75 percentile, and whiskers indicate minimum and maximum measurements. ( j ) Representative image showing high-level SOX2-positive cells (green), TECs (CD31, red) and nuclear chromatin (DAPI, blue). White dotted line indicates tumour–stroma interface. Scale bar, 20 μm. Full size image Elevated expression levels of Vegfa and Nrp1 suggested that Sox2-positive cells might be located in close proximity to tumour endothelial cells as previously reported for CD34-positive TICs, which express elevated levels of Nrp1, Vegfa, as well as Sox2 (ref. 40 ). To test this hypothesis, we measured the closest distance between basal SCC cells with high SOX2 expression and CD31-positive tumour endothelial cells by quantitative immunofluorescence microscopy. Our measurements revealed that SCC cells, which are located at the tumour–stroma interface and express high levels of SOX2, are often found in clusters located in close proximity to CD31-expressing tumour endothelial cells ( Fig. 3i,j ). SOX2 controls NRP1 expression and SCC growth Nrp1/Vegfa signalling is critical for tumour growth in murine SCC where it promotes cell proliferation, survival and symmetric self-renewal [40] , [41] . To investigate whether NRP1 expression is dependent on SOX2 function in human SCC, we first measured the relative expression levels of NRP1 in control and SOX2-depleted human SCC cells. qRT–PCR revealed significantly reduced NRP1 expression in shSOX2-depleted human SCC cells compared with controls ( Fig. 4a ). In addition, SOX2 was significantly enriched at the NRP1 locus as measured by quantitative ChIP–PCR analyses ( Fig. 4b ). These data together with Nrp1’s previously described role in murine SCCs suggested NRP1 as one possible molecular target responsible for SCC initiation and growth in human SCCs. 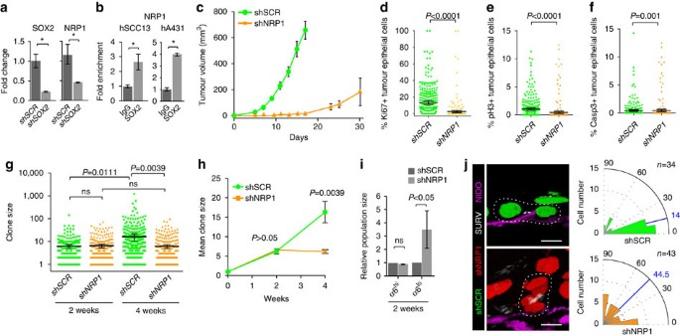Figure 4: NRP1 expression is regulated by SOX2 and required for SCC growth. (a) qRT–PCR analysis of SOX2 and NRP1 on human SCC13 cells transduced with shSCR and shSOX2. (b) qRT–PCR analyses on chromatin samples from cultured human SCC13 and A431 cells after immunoprecipitation with anti-Sox2 and IgG control antibodies. (a,b) Bar graphs show mean with error bars indicating ±s.d (n=3, *P<0.05 Student’st-test). (c) Tumour growth curves of A431 cells grafted onto Nude recipient mice after transduction with shNRP1;H2B-RFP or shSCR;H2B-GFP. Data are represented as mean with error bars indicating ±s.e.m. (n=6, *P<0.05, Student’st-test). (d–f) Quantitative analysis of proliferative Ki67 (d), mitotic phospho-Histone H3(Ser10) pH3 (e) and apoptotic activated Caspase-3 (Casp3)- (f) positive cells in shNRP1;H2B-RFP or shSCR;H2B-GFP-transduced A431 xenografts. Scatter plots illustrate the percentage of infected parenchymal cells that are positive for the respective marker inn>200 microscopic fields. Horizontal bars indicate mean±95% confidence interval (CI). (*P<0.05, Mann–Whitney non-parametrict-test). (g,h) Analysis of clonal growth competition assays at 2 and 4 weeks after intradermal transplantation when 1–2% of A431 cells have been transduced with shNRP1;H2B-RFP and shSCR;H2B-GFP (n=6). (g) Scatter plots illustrate clone size distributions. Horizontal lines represent mean with error bars indicating±95% CI. (h) Line graphs show average clone size as a function of time (±s.e.m.). (g,h)P-values were obtained by Mann–Whitney non-parametrict-tests. (i) Flow cytometric analyses of basement membrane-associated clones (integrin α6hi) in clonal competition assays 2 weeks after transplantation. Bar graphs show mean population size of shNRP1;H2B-RFP- and shSCR;H2B-GFP-expressing cells within the α6-integrin-high and α6-integrin-low gates. Error bars indicate ±s.d. (n=6, *P<0.05, Student’st-test). (j) Projections of representative three-dimensional immunofluorescence micrographs (left) and radial histograms (right) indicating the orientation of basal cell divisions relative to the tumour–stroma interface in shSCR;H2B-GFP control (top,n=34) and shNRP1;H2B-RFP (bottom, n=43) human A431 SCC grafts. Survivin marks the spindle mid-body (SURV, white) and Nidogen (NIDO, magenta) demarcates the basement membrane. Scale bars, 10 μm. Blue lines indicate median division angles. Statistical significanceP<0.01 was determined by Mann–Whitney non-parametrict-test. Figure 4: NRP1 expression is regulated by SOX2 and required for SCC growth. ( a ) qRT–PCR analysis of SOX2 and NRP1 on human SCC13 cells transduced with shSCR and shSOX2. ( b ) qRT–PCR analyses on chromatin samples from cultured human SCC13 and A431 cells after immunoprecipitation with anti-Sox2 and IgG control antibodies. ( a , b ) Bar graphs show mean with error bars indicating ±s.d ( n =3, * P <0.05 Student’s t -test). ( c ) Tumour growth curves of A431 cells grafted onto Nude recipient mice after transduction with shNRP1;H2B-RFP or shSCR;H2B-GFP. Data are represented as mean with error bars indicating ±s.e.m. ( n =6, * P <0.05, Student’s t -test). ( d – f ) Quantitative analysis of proliferative Ki67 ( d ), mitotic phospho-Histone H3(Ser10) pH3 ( e ) and apoptotic activated Caspase-3 (Casp3)- ( f ) positive cells in shNRP1;H2B-RFP or shSCR;H2B-GFP-transduced A431 xenografts. Scatter plots illustrate the percentage of infected parenchymal cells that are positive for the respective marker in n >200 microscopic fields. Horizontal bars indicate mean±95% confidence interval (CI). (* P <0.05, Mann–Whitney non-parametric t -test). ( g , h ) Analysis of clonal growth competition assays at 2 and 4 weeks after intradermal transplantation when 1–2% of A431 cells have been transduced with shNRP1;H2B-RFP and shSCR;H2B-GFP ( n =6). ( g ) Scatter plots illustrate clone size distributions. Horizontal lines represent mean with error bars indicating±95% CI. ( h ) Line graphs show average clone size as a function of time (±s.e.m.). ( g , h ) P -values were obtained by Mann–Whitney non-parametric t -tests. ( i ) Flow cytometric analyses of basement membrane-associated clones (integrin α6 hi ) in clonal competition assays 2 weeks after transplantation. Bar graphs show mean population size of shNRP1;H2B-RFP- and shSCR;H2B-GFP-expressing cells within the α6-integrin-high and α6-integrin-low gates. Error bars indicate ±s.d. ( n =6, * P <0.05, Student’s t -test). ( j ) Projections of representative three-dimensional immunofluorescence micrographs (left) and radial histograms (right) indicating the orientation of basal cell divisions relative to the tumour–stroma interface in shSCR;H2B-GFP control (top, n =34) and shNRP1;H2B-RFP (bottom, n=43) human A431 SCC grafts. Survivin marks the spindle mid-body (SURV, white) and Nidogen (NIDO, magenta) demarcates the basement membrane. Scale bars, 10 μm. Blue lines indicate median division angles. Statistical significance P <0.01 was determined by Mann–Whitney non-parametric t -test. Full size image To test whether NRP1 function is critical to skin carcinogenesis in human, we first compared the growth kinetics of shSCR-GFP and shNRP1-RFP in our xenotransplantation model. Similar to SOX2, NRP1 depletion resulted in 40% reduced SCC initiation, spontaneous regression of one tumour and significantly delayed growth kinetics of the remaining transplants ( Fig. 4c ). Consistent with the slower tumour growth, we measured significantly reduced proliferation ( Fig. 4d,e ), while apoptosis rates were comparable between shNRP1- and shSCR-expressing tumours ( Fig. 4f ). Likewise, quantitative lineage trace analyses of clonally transduced human SCCs revealed no significant differences in the initial growth followed by the depletion of shNRP1-RFP knockdown clones compared with shSCR-GFP controls, mirroring the growth behaviour of SOX2-depleted SCC cells ( Fig. 4g,h ). Intriguingly, flow cytometric analyses of our clonal competition experiments revealed a subtle decrease in the relative number of NRP1-depleted SCC cells expressing high levels of α6 integrin, while the population of NRP1-deficient cells expressing low levels of α6 integrin was significantly increased ( Fig. 4i ). These data suggest that NRP1-depleted clones might also differentiate more rapidly than SCR controls within the same tumour. This observation is consistent with previous reports where Nrp1 functions to promote self-renewing cell divisions along the tumour–stroma interface in murine SCCs [40] . To test whether this function of Nrp1 is conserved in human SCCs, we stained our xenografts with the spindle mid-body marker Survivin and the extracellular matrix marker Nidogen, and measured the orientation of cell divisions relative to the tumour–stroma interface of test (shNRP1-RFP) and control (shSCR-GFP) cells within the same tumour. Control basal SCC cells divided predominantly along the tumour–stroma interface, while the orientation of NRP1-depleted basal SCC cell divisions appeared randomized ( Fig. 4j ). Given the direct links between SOX2 and NRP1 expression, we wondered whether SOX2 expression correlates with oriented cell divisions along the tumour–stroma interface. We first stained human SCC xenografts with the spindle mid-body marker Survivin and measured the orientation of basal, SOX2-positive and SOX2-negative cell divisions in late mitosis. We observed that SOX2-positive cells divided predominantly parallel to the basement membrane, whereas the division axis of the rare, SOX2-negative basal SCC cells was randomized ( Fig. 5a,b ). A similar distribution was observed in primary mouse SCCs where Sox2-negative cells are more common ( Fig. 5c ). To functionally probe this correlation and test whether SOX2 is indeed required to direct the orientation of basal SCC cells, we measured the division axis in shSCR-GFP control and shSOX2-RFP knockdown clones with respect to the tumour–stroma interface. Our measurements revealed that basal cells within control clones divided primarily in parallel to their underlying stroma, whereas the division axis in basal SOX2 knockdown cells was randomized in both human ( Fig. 5d,e ) and mouse ( Fig. 5f ) SCC grafts. These results support the hypothesis that Sox2 expression biases TICs to divide along the tumour–stroma interface, thereby expanding the undifferentiated and proliferative tumour fraction/compartment. 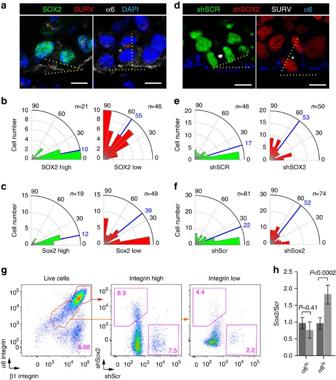Figure 5: SOX2 expression promotes TIC divisions along the tumour–stroma interface. (a) Confocal sections of human SCCs stained with SOX2 (green), Survivin (SURV, red), α6-integrin (α6, white) and DAPI (blue). Scale bars, 10 μm. (b,c) Radial histograms indicating the orientation of basal cell divisions relative to the tumour–stroma interface expressing high (green) or low (red) levels of SOX2 in human (b) and mouse (c) SCCs. Blue lines indicate median division angles. (d) Projections of representative three-dimensional immunofluorescence micrographs of shSCR;H2B-GFP and shSOX2;H2B-RFP clones in A431 xenografts stained with Survivin (SURV, white) and α6-integrin (blue). Scale bars, 10 μm. (e,f) Radial histograms describe the orientation of basal cell divisions relative to the tumour–stroma interface in shSCR;H2B-GFP (green) and shSOX2;H2B-RFP (red) clones in human (e) and mouse (f) SCC transplants. Blue lines indicate median division angles. (g,h) Flow cytometric analyses of shSCR;H2B-GFP and shSOX2;H2B-RFP clonal competition assays 2 weeks after transplantation. (g) Scatter plots illustrate the relative abundance of shSCR;H2B-GFP and shSOX2;H2B-RFP cells within the α6/β1-integrin high and low gates. (h) Bar graphs show mean population size of shSOX2;H2B-RFP- and shSCR;H2B-GFP-expressing cells within the α6-integrin-high and α6-integrin-low gates with error bars indicating ±s.d (n=6, *P<0.05, Student’st-test). Figure 5: SOX2 expression promotes TIC divisions along the tumour–stroma interface. ( a ) Confocal sections of human SCCs stained with SOX2 (green), Survivin (SURV, red), α6-integrin (α6, white) and DAPI (blue). Scale bars, 10 μm. ( b , c ) Radial histograms indicating the orientation of basal cell divisions relative to the tumour–stroma interface expressing high (green) or low (red) levels of SOX2 in human ( b ) and mouse ( c ) SCCs. Blue lines indicate median division angles. ( d ) Projections of representative three-dimensional immunofluorescence micrographs of shSCR;H2B-GFP and shSOX2;H2B-RFP clones in A431 xenografts stained with Survivin (SURV, white) and α6-integrin (blue). Scale bars, 10 μm. ( e , f ) Radial histograms describe the orientation of basal cell divisions relative to the tumour–stroma interface in shSCR;H2B-GFP (green) and shSOX2;H2B-RFP (red) clones in human ( e ) and mouse ( f ) SCC transplants. Blue lines indicate median division angles. ( g , h ) Flow cytometric analyses of shSCR;H2B-GFP and shSOX2;H2B-RFP clonal competition assays 2 weeks after transplantation. ( g ) Scatter plots illustrate the relative abundance of shSCR;H2B-GFP and shSOX2;H2B-RFP cells within the α6/β1-integrin high and low gates. ( h ) Bar graphs show mean population size of shSOX2;H2B-RFP- and shSCR;H2B-GFP-expressing cells within the α6-integrin-high and α6-integrin-low gates with error bars indicating ±s.d ( n =6, * P <0.05, Student’s t -test). Full size image Indeed, we counted significantly fewer undifferentiated, α6 and β1 integrin-expressing cancer cells in Sox2-depleted clones when compared with Scr controls ( Supplementary Fig. 8k ). In addition, sensitive flow cytometry assays corroborated this observation, as they detected a small reduction in the relative portion of undifferentiated α6-high SCC cells and a significant increase in post mitotic, differentiating α6-low SCC cells even at 2 weeks after transplantation, when no significant differences in total clone size were detected ( Fig. 5g,h ). Together, these data suggest that Sox2 enhances TIC self-renewal and suppresses their differentiation, thereby promoting geometric growth within SCCs [42] . Our study on cutaneous SCC, a paradigm for hierarchically organized cancers, provides important insights about the regulation of cancer cells with tumour initiating potential and their consequences for tumour growth. Cutaneous SCCs are, similar to normal skin epithelium, sustained by stem cells that self-renew and differentiate into progeny without long-term proliferative potential [42] . Although, TICs and normal skin epithelial stem and progenitor cells share some similarities, including the following: their close association with the underlying stroma; their elevated expression of cell surface markers α6 integrin, β1 integrin and CD34; their clonogenic potential in culture; and their regenerative capacity in vivo , our differential gene expression analyses identified a gene expression signature that distinguishes TICs from HFSCs [14] , [20] , [21] , [43] . Surprisingly, transcription factors that specify HFSC and sustain their long-term self-renewing potential are not detected in TICs of SCC. Instead, a tumour-specific transcriptional programme, not expressed in normal skin epithelial cells, becomes established de novo as SCCs initiate and progress ( Fig. 1 ). This programme, which specifies TICs and distinguishes them from normal skin epithelial stem and progenitor cells both molecularly and functionally, is expressed in both mouse and human SCCs. As part of this tumour-specific transcriptional programme, we discovered Sox2 as a novel, functional marker for TICs in mouse and human SCCs. Although tightly repressed in normal skin epithelium and dispensable for skin epithelial homeostasis, Sox2 activity is critical for tumour initiation, maintenance and SCC growth in mouse and human. The expression of Sox2 during the course of carcinogenesis correlates with a loss of the repressive H3K27me3 chromatin mark at the Sox2 promoter, while its copy number was unaffected ( Supplementary Fig. 5 ). Intriguingly, the reduction of H3K27me3 appears to be locus specific rather than global, as Polycomb Repressive Complex components are expressed and active. Although the molecular mechanisms leading to the de-repression of Sox2 remain to be identified in cutaneous SCCs, a similar locus-specific de-repression resulting in de novo Sox2 expression in synovial sarcoma had been linked to the disruption of mSWI/SNF (BAF) complexes [44] . Once expressed, Sox2 becomes essential for SCC growth and maintenance. Our findings therefore suggest the feasibility of therapies that directly aim at cancer cells with tumour initiating potential, while leaving normal stem and progenitor cells unaffected. The successful development of such therapies, however, will require a comprehensive understanding of the circuitry that enables and sustains Sox2 expression in TICs of SCC, in addition to the identification of lineage-specific transcription factors that partner with Sox2 to sustain its activity in SCC TICs. Although our current study focuses on a subset of Sox2 target genes that are common between TICs in SCC and ESCs, it remains to be defined how Sox2 regulates the expression of these genes. This is important because the Sox2 partners Oct4 and Nanog, which are critical for its function in ESCs, are not expressed in SCC TICs ( Supplementary Fig. 3 ) [20] . Indeed, several novel Sox2-binding partners have been identified in human head and neck SCCs [45] , directing Sox2 activity to numerous genomic loci, where it can function as both a transcriptional activator as well as a repressor [46] . Nrp1 has surfaced together with several other pro-angiogenic factors as direct Sox2 target genes with the highest differential expression between TICs and skin epithelial stem and progenitor cells. Importantly, Nrp1 was not only a Sox2 target in mouse but also in human. In addition to Nrp1, Vegfa and the Egf-receptor ligands tumour growth factor-α and Epiregulin are also highly expressed in TICs, while they are not detected in HFSCs ( Supplementary Fig. 1c ). Our data therefore suggest a critical role for Sox2 in promoting a synergistic autoregulatory feedback loop between Nrp1/Vegf and Egfr signalling, which promotes proliferation and cell survival to drive rapid SCC growth [40] , [41] , [47] . Combined inhibition of Egfr and Vegf signalling in skin epithelial cells prevents the initiation of skin tumours [41] . Consistent with this report, we find a 50% reduction in the tumour initiating potential of Sox2-depleted tumours. Intriguingly, the shSox2-RFP transduced tumours, which did initiate, were often comprised of both transduced and untransduced SCC cells, suggesting the possibility that growth factors secreted from Sox2-positive tumour epithelial cells may have supported the growth of Sox2-depleted tumour cells. Nevertheless, proliferation rates were significantly reduced as previously reported for SCCs where Nrp1/Vegf signalling was compromised [40] , [41] and apoptosis rates were significantly increased consistent with compromised Egfr signalling in SCCs [47] . Interestingly, Sox2 depletion in single cell clones also affected the rate of tumour cell clone size expansion in human and mouse, indicating that Sox2-positive clones expand geometrically, whereas SOX2 knockdown clones appeared to expand via linear growth kinetics ( Fig. 2f,g and Supplementary Fig. 8f,g ). A similar result was obtained in human SCCs, when NRP1 was depleted at the clonal level ( Fig. 4g,h ). This growth difference could be simply explained by the reduced proliferation and apoptosis rates. However, it is intriguing to speculate that SOX2 or NRP1-depleted TICs could change the mode rather than the rate of cell division. In normal epidermis, the progenitor cell pool can expand by symmetric cell divisions in the basal layer that are parallel in respect to their underlying basement membrane, while perpendicular divisions enable an asymmetric lineage choice, which maintains an uncommitted and proliferative basal daughter cell, in addition to an apical daughter that commits to squamous differentiation [48] , [49] . Indeed, symmetric and asymmetric cell divisions have also been described in basal cells of murine SCCs, where the division axis was dependent on Nrp1 function [40] . In analogy to these studies, we observed differences in the orientation of dividing SOX2-positive and SOX2-negative SCC cells with respect to the tumour–stroma interface. Although our data support the hypothesis that SOX2 and NRP1 promote the division and expansion of TICs along the tumour–stroma interface to expand the proliferative SCC cell pool, further studies including the reconstruction and measurement of TIC divisions in three dimensions and the identification of cell fate determinants, which differentially segregate between daughter cells on cytokinesis, are required before the divisions can be defined as either symmetric or asymmetric. To date, mechanisms controlling self-renewal and differentiation are only beginning to emerge. Still, the mode by which TICs divide may be critical for therapy resistance and therapy design [50] . Therefore, our observation that division orientation and geometric expansion in clonal trace experiments depend on SOX2/NRP1 function in both mouse and human SCCs provide a starting point to further investigate the links between cell division and differentiation in skin carcinogenesis. Taken together, our data suggest that Sox2 functions as a pivotal molecule in SCCs, as it acts as an integration point of developmental and oncogenic signalling mechanisms. Sox2 expression not only renders TICs self-sufficient for essential mitogenic stimuli, it also provides critical pro-angiogenic cues that ensure the blood supply and waste disposal for a rapidly expanding tumour—thereby affecting several hallmarks of cancer [51] . Constructs and RNAi All shRNAs were obtained from the Mission TRC-1 mouse and human library (Sigma), cloned into pLKO.1 (Addgene 8453) and subsequently cloned into pLKO Histone H2B-mRFP1 (Addgene 26001) or pLKO Histone H2B-GFP (Addgene 25999) [34] , or cloned directly into pLKO Tet-on puro (Addgene 21915) [52] . pLKO-no stuffer-PGK-mSox2-3X Flag was generated as follows: (1) mSox2 was amplified by PCR from FU-CRW-mSox2-RFP using primers 5′-atgcatAAGCTTgtatggtcccgggggcagcg-3′ and 5′-atgcatAGATCTtcacatgtgcgacaggggca-3′, and then digested with Hind III and Bgl II. The PCR product was ligated with 3XFLAG-CMV10, digested with Hind III and Bgl II, to generate 3xFlag-mSox2-CMV10. (2) mSox2 was PCR amplified from 3xFlag-mSox2-CMV10 using primers 5′-atgcatACCGGTaccatggtatggtcccgggggca-3′ and 5′-atgcatCTCGAGcatgtgcgacaggggcagtg-3′, and then the PCR product and PQCXIX-MCS-3xFlag-IRES-tomato were digested with Age I and Xho I, and ligated to generate PQCXIX-mSox2-3xFlag-IRES-tomato. (3) PQCXIX-mSox2-3xFlag-IRES-tomato and pLKO no stuffer PGK MCS were digested with Bam HI and Blp I, and mSox2-3xFlag was subcloned into pLKO no stuffer-PGK-MCS to generate pLKO-no stuffer-PGK-mSox2-3X Flag. The following shRNAs were used: shScramble (SHC002), shSox2 (TRCN0000424718, TRCN0000085748, TRCN0000231643 and TRCN0000257314) and shNRP1 (TRCN0000322980). For full hairpin sequences, see Supplementary Table 1 . Cell culture All primary cell lines were maintained as previously described [53] , [54] , except for human squamous cell line SCC-13, which was grown in 1.5 μM calcium (high-calcium medium) and human cell line A431, which was grown in DMEM with 10% fetal bovine serum (FBS). Human head and neck SCC cell lines were cultured in P medium (DMEM:F12 (3:1), sodium bicarbonate (Sigma), L -glutamine (Invitrogen) and Pen/Strep solution (Invitrogen)) with 10% FBS). Human cell lines were obtained from ATCC (A431) or Harvard Skin Disease Research Center Cell Culture Core [27] , and primary murine cell lines were tested for mycoplasma contamination (mouse essential virus panel, Charles River Research Animal Diagnostic Services). For stable cell line generation, lentivirus was produced by Lipofectamine 2000 (Invitrogen) transfection of 293FT cells (Invitrogen) with pLKO shRNA-carrying plasmid and helper plasmids pMD2.G and psPAX2 (Addgene plasmid 12259 and 12260, respectively). 293FT cells were maintained in media consisting of 75% D10 media (DMEM (Gibco), 0.075% sodium bicarbonate, 1% L -glutamine and Pen/Strep solution (Invitrogen), 10% FBS, 1 mM sodium pyruvate (Invitrogen)) and 25% OptiMem Mix (Opti-MEM (Invitrogen) and 10% FBS). Viral supernatant was collected 36 h and 60 h after transfection, and filtered through a 0.22-μm filter. For viral infections, 10,000 cells were plated per well in 6-well plate and incubated with lentiviral supernatant in the presence of 31 μg ml −1 of polybrene and spun at 1,100 g for 30 min at 37 °C. Infected cells were FACS-sorted 60 h post infection and used in analyses of in vivo tumour growth (whole tumour and clonal competition) and in vitro clonal competition. For tumour growth assays, FACS isolations were performed on a BD FACSAria II equipped with 488, 633, 405, 562 and 355 nm lasers. Cells were gated on live, single cells, and sorted for either GFP+ or RFP+ (shRNA-carrying) cell populations. Sorted cells were suspended in 50% Matrigel (356237; BD) diluted with F medium at a concentration of 10,000 (murine) or 50,000–100,000 (human) cells per injection and injected intradermally into Nude (NU/NU [088] Charles River) recipient mice. For clonal competition assays, both viruses (Scr-GFP and Sox2-RFP) were produced in the same well by using equal amounts of each shRNA-carrying plasmid. Infected cells were analysed before injection to determine RFP/GFP ratios using a BD LSR II. Antibodies, immunohistochemistry and imaging Unfixed tumours were embedded in OCT (Tissue Tek). Frozen sections were cut to a thickness of 12–30 μm on a Leica cryostat and mounted on SuperFrost Plus slides (Fisher). Slides were air-dried for 10 min, then fixed for 5–10 min with 4% formaldehyde (28908, Thermo Scientific), rinsed with PBS, permeabilized with 0.1% Triton X-100 in PBS for 15 min, then blocked for 1 h in gelatin block (5% normal donkey serum, 1% BSA, 2% gelatin, 0.2% Triton X-100 in PBS) or NDS/NGS block (5% normal donkey serum, 5% normal goat serum, 0.2% Triton X-100 in PBS) and incubated in primary antibody diluted in blocking buffer at 4 °C overnight. After washing with PBS, secondary antibodies, conjugated to Alexa 488, fluorescein isothiocyanate, Alexa 568, DyLight 649, DyLight 405 and Hoechst 33342 (83218, AnaSpec) were diluted in blocking buffer and incubated with the slides for 1 h at room temperature (RT). After washing, slides were mounted in ProLong Gold (Invitrogen) or Vectashield (H-1400, Vector Laboratories). Imaging was performed on a Nikon Eclipse TiE Microscope, Leica TCS SP5 II Confocal Microscope, Zeiss LSM510 Confocal Microscope or Zeiss LSM780 Confocal Microscope. Image stacks were visualized in Volocity 6.0. For Survivin and Sox2 co-stainings on primary mouse and human xenograft SCC tumours, the same protocol was followed, except for the following: sections were incubated overnight with rabbit anti-Sox2, washed, stained with secondary anti-rabbit Alexa 488, washed and incubated with rabbit anti-survivin and rat anti-CD104/β4 (mouse samples only) or rat anti-CD49f/α6-PerCP-Cy5.5 (human samples only) overnight, washed and incubated with secondary anti-rabbit Alexa 568, anti-rat DyLight 649 and Hoechst, washed and mounted in ProLong Gold. For detailed list of antibodies and dilutions, see Supplementary Table 2 . Human tissue microarray and paraffin SCC and metastases stainings Primary human SCC specimens have been de-identified and supplied by NYU’s tissue acquisition and banking service. Human skin squamous cancer tissue microarray (SK802a, US Biomax) was dewaxed and hydrated (2 × xylene, 2 × 100% ethyl alcohol, 2 × 95% ethyl alcohol, 1 × 70% ethyl alcohol and 1 × 50% ethyl alcohol for 3 min each). After rinsing in PBS, slides were placed into a water bath (98 °C for 20 min) in sodium citrate buffer (10 mM sodium citrate, pH 6.0) for heat-induced antigen retrieval. Endogenous peroxidase activity was blocked using BloxALL (SP-6000, Vector Laboratories) for 10 min at RT after wash in PBS. Following washing, slides were blocked in NHS block (0.3% Triton X-100, 1% BSA, 5% normal horse serum in PBS) for 30 min at RT. Primary antibody was diluted in NHS blocking buffer and slides incubated at 4 °C overnight. Slides were washed with 0.3% Triton X-100 in PBS and incubated with biotinylated secondary anti-rabbit IgG (H+L) for 30 min at RT. After final washes, slides were incubated with ABC solution (PK-4000, Vector Laboratories) for 30 min at RT. Following washes, staining was developed by incubating with ImmPACT DAB (SK-4105, Vector Laboratories) for 2–10 min at RT. Reaction was stopped by washing with ddH 2 O. Slides were dehydrated (1 × 50% ethyl alcohol, 1 × 70% ethyl alcohol, 1 × 95% ethyl alcohol, 2 × 100% ethyl alcohol and 2 × xylene for 3 min each) and mounted with Permount (SP-15-100, Fisher Scientific). A detailed list of antibodies and their working concentrations can be found in Supplementary Table 2 . Genomic meta analyses Differential gene expression analyses between CSCs, EPI and HFSCs (GSE29328) has been analysed in Gene Pattern software as previously described [20] . Average expression values across 16 independent CSC populations and replicate HFSC or EPI populations has been computed in MATLAB and presented as scatter plots. Transcription factors with the highest differential expression values in CSCs and HFSCs have been indicated as red and green dots, respectively. Pre-computed Sox2 peaks obtained from GEO repository accession number GSE11431 (series GSM288347) were converted from assembly version mm8 to assembly version mm10 using UCSC Genome Browser liftover utility [55] and used for our analyses. Read alignments to human assembly version hg18 were downloaded from GEO (accession series GSM456570) and peaks were computed using MACS [56] version 1.4 with default parameters, except for using a fragmentation size of 400 bp. Peaks were then converted to human assembly version hg19 using UCSC Genome Browser liftover utility. Quantitative reverse-transcription PCR For culture experiments, cells were grown at 4%O 2 , 7% CO 2 and serum-starved 24 h before harvesting. mRNA was isolated using Qiazol (Qiagen) and Direct-zol RNA Mini Prep (R2052, Zymo Research), or Absolutely RNA Nanoprep Kit (400753, Agilent Technologies). Samples were quantified using a Nanodrop spectrophotometer (Thermo Scientific). Complementary DNA was synthesized from 300 ng to 1.5 μg of total RNA using SuperScript VILO with random primers (Invitrogen) or SuperScript III First-Strand Synthesis System (Invitrogen) with oligo(dT) primers. qRT–PCR was performed with Absolute Blue QPCR SYBR Green Mix plus ROX Vial Kit (AB-4166, Thermo Scientific) on a MyiQ2 (BioRad), or with LightCycler DNA Master SYBR Green I reagents (Roche) on a Light Cycler 480 (Roche). Measurements were recorded in duplicate or triplicate. Differences between samples and controls were calculated based on the 2 −ΔΔCT method and normalized to Rplp0 (mouse) or RPLP0 (human). For detailed list of primer sequences, see Supplementary Table 3 . Chromatin immunoprecipitation–PCR For chromatin immunoprecipitation, cells were grown at 4%O 2 , 7% CO 2 and serum-starved 24 h before harvesting. Cells were fixed in fixation buffer (1% formaldehyde, 10 mM HEPES pH7.6, P low calcium media (50 μM calcium, DMEM:F12 {3:1} without calcium) (special order, Gibco catalogue number 90-5010EA), sodium bicarbonate, L -glutamine and Pen/Strep solution), lysed using a series of lysis buffers (lysis buffer I (50 mM HEPES pH7.6, 140 mM NaCl, 1 mM EDTA, 10% glycerol, 0.5% NP-40 and 0.25% Triton X-100 in ddH 2 O), lysis buffer II (10 mM Tris–HCl pH8.0, 200 mM NaCl, 1 mM EDTA and 0.5 mM EGTA in ddH 2 O) and lysis buffer III (10 mM Tris–HCl pH 8.0, 1 mM EDTA, 0.5 mM EGTA and 0.5% N -lauryl sarcosine in ddH 2 O)) with cOmplete, Mini, EDTA-free protease inhibitor tablets (04693159001, Roche). Chromatin was sonicated to 200–500 base pair fragments using a Diagenode Bioruptor (Diagenode) employing a 30 s on/off regime. For Sox2 ChIP experiments on mouse and human SCC cell extracts, chromatin immunoprecipitation was performed according to the manufacturer’s instructions using the EZ-Magna ChIP kit (Millipore). Chromatin (40 or 80 μg per immunoprecipitation) was immunoprecipitated with 2 or 4 μg mouse monoclonal anti-Sox2 antibody (17–656, Millipore) or control normal mouse IgG (17–656, Millipore) at 4 °C overnight. For H3K27me3 ChIP experiments, ChIP assay was performed using 10 6 cells per immunoprecipitation with 25 μl Dynabeads Magnetic Protein G (12321D, Invitrogen) and 5 μg anti-H3K27me3 (ab6002, Abcam) or control normal mouse IgG/IgG2b (sc-2025, Santa Cruz). qRT–PCR was performed with the Absolute Blue QPCR SYBR Green Mix plus ROX Vial Kit (AB-4166, Thermo Scientific) on a MyiQ2 (BioRad), or FastStart Universal SYBR Green Master Mix (4913914001, Roche) on a StepOnePlus (Life Technologies). Relative binding was calculated with the 2 −ΔΔCT method and normalized to input. For detailed primer sequences, see Supplementary Table 4 . SOX2 copy gene number Genomic DNA was isolated using DNeasy Blood & Tissue Kit (69504, Qiagen). SOX2/Sox2 copy number was analysed using the TaqMan copy number assay from Applied Biosystems (kit 4371355) and the TaqMan probe Hs 02753059 or Mn00549969. SOX2/Sox2 copy number was calculated relative to TERT/RNaseP or Tert/Tfrc expression, using the CopyCaller Software v2.0 from Applied Biosystems. Western blotting Cell lysates were prepared using RIPA buffer (150 mM sodium chloride, 0.1% Triton-X 100, 0.5% SDS and 50 mM Tris pH 8 in ddH 2 O) with complete Mini EDTA-free protease inhibitor tablets (04693159001, Roche). Protein concentrations were determined following the instructions of Pierce BCA Protein Assay Kit (23225, Pierce). Lysates were boiled with 3 × Laemmli buffer (6% SDS, 15% β-mercaptoethanol, 30% glycerol, 0.006% bromophenol blue, 0.188 M Tris–HCl) for 10 min at 95 °C. Protein ladder used was Full-Range Rainbow Molecular Weight Markers (RPN800, GE Healthcare). For murine samples, 30 μg of protein was loaded per lane. For human samples, 10–120 μg of protein was loaded per lane. Gel electrophoresis was performed using a 10 or 12% Bis-Tris gel run for 75–150 min at 120 V, gel was transferred for 1 h at 4 °C at 100 V to a 0.45 μm nitrocellulose membrane (Whatmann) and transfer was assessed by Ponceau S staining (0.1% (w/v) Ponceau S in 5% (v/v) acetic acid). Membranes were blocked with 5% non-fat dry milk in TBST, then incubated with primary antibodies diluted in blocking buffer or antibody dilutent (5% (w/v) BSA in TBST (TBS with 0.1% Tween-20)) overnight at 4 °C with gentle agitation. Membranes were rinsed with TBST before incubating with horseradish peroxidase-conjugated secondary antibodies diluted in blocking buffer for 1 h at RT. Membranes were washed with TBST, then with TBS before incubating with the Luminata Classico or Crescendo Western horseradish peroxidase Substrate (WBLUC0500 or WBLUR0500, Millipore) and exposed to X-ray film (F-9024-8 × 10, GeneMate) using a Kodak X-Omat 2000A Processor. For detailed list of antibodies and dilutions, see Supplementary Table 2 . Full scans of western blotting films are provided in Supplementary Fig. 9 . Tumour isolation and flow cytometry Tumours from murine allografts and human xenografts were isolated as previously described [20] . Briefly, after separating tumours from normal skin, blood vessels and connective tissue, tumours were minced and incubated with 0.25% collagenase (C2670, Sigma) in HBSS (Gibco) for 60 min at 37 °C shaking. During the last 10 min of collagenase digestion, 62.5 U ml −1 DNaseI (LS002138, Worthington) was added. The cell suspension was filtered through 70 and 40 μm cell strainer, where tissue remaining in filters was digested an additional 10 min with 0.25% trypsin (Invitrogen) at 37 °C shaking and strained again. Cell suspensions were diluted in wash buffer (2% chelexed FBS in DPBS) and pelleted at 300 g for 10 min. For human foreskin isolations, fat layer was removed from samples and incubated with the dermis-side down, in dispase (354235, BD Biosciences) overnight at 4 °C. Epidermis was physically separated from the dermis, and rinsed in PBS followed by a 10 min incubation in trypsin at 37 °C. Tissue was dissociated and filtered through a 70- and 40-μm cell strainer. Isolated cells were plated on 3T3 feeder cell layer in E medium with 15% Ca 2+ -free FBS, 300 μM calcium and Antibiotic-Antimycotic (15240112, Invitrogen). For flow cytometry, cell suspensions were stained for 30 min on ice (for a detailed list of antibodies and dilutions see Supplementary Table 2 ) and DAPI (4′,6-diamidino-2-phenylindole; D1306, Invitrogen) was used for live/dead cell exclusion. FACS analyses were performed on a BD LSRII equipped with 488, 642, 407, 355 and 562 nm lasers. Flow cytometry data analysis was carried out using FlowJo. For pre-injection clonal competitions, RFP+ and GFP+ cell populations were gated on live, single cells. For post-injection clonal competitions, RFP+ or GFP+ integrin hi and integrin low cell populations were gated on live, single, RFP+ or GFP+ cells (lineage marker) followed by α6 hi β1 hi (basal) and α6 low β1 low (suprabasal) cells. Epidermal stem and progenitor populations and HFSCs were sorted from single, live (DAPI), lineage-positive (K14-H2BGFP) [11] , CD49f-positive cells as the Sca1- and CD34-positive cell populations, respectively. Dermal papillae cells were isolated from single, live (DAPI), lineage-positive (Lef1-RFP [57] and Itga9-positive cell populations [58] . Mice Female 6-week-old Nude (NU/NU [088] Charles River) mice were used for orthotypic transplantations and xenograft studies. Tumours were detected by palpation, measured using a digital caliper and tumour volume was calculated ( , where l=length in mm and w=width in mm). Mice were injected intraperitoneally with 5-bromo-2′-deoxyuridine (Invitrogen 5 μl mg −1 of weight) 8 h before sacrificing. For inducible RNA interference (RNAi)-mediated knockdown in vivo , mice were placed on doxycycline-containing (200 mg) diet after tumours were established, while control mice remained on a normal diet. Tumour volumes were calculated at the time mice where placed on doxycycline and this volume served as the baseline to calculate the fold change of tumour volume over time in treated and control mice. All animal experiments were performed in accordance with the guidelines and approval of the Institutional Animal Care and Use Committee at New York University Langone Medical Center. Measurements, quantification, graphing and statistics All experiments were carried out single blinded, except for quantification of division axis in Sox2/SOX2 high and low cells, and assessment of SOX2 expression in patient SCC tissue microarrays, which were double blinded. All RNAi-mediated knockdown experiments in vivo and in vitro were repeated three independent times with biological replicates. All quantitative data were collected from experiments performed in at least triplicate, and expressed as mean±s.d., 95% confidence interval, min/max or s.e.m. Differences between groups were assayed using unpaired or paired two-tailed Student’s t -test, or Mann–Whitney test (proliferation and apoptosis quantifications, clonal size distributions and division axis) using Prism 6 (GraphPad Software). Box-and-whisker plots are used to describe the entire population without assumptions about the statistical distribution. Significant differences were considered when P <0.05 as indicated by asterisks. For clonal competition assays, population sizes were determined by counting RFP+ or GFP+ cells. Integrin-high clones were defined as at least one RFP+ or GFP+ cell was located at the tumour–stroma interface (as indicated by CD104/β4 or CD49f/α6 staining) per clone. For proliferation and apoptosis quantifications, pictures were acquired at × 20 magnification and deconvolved, before Ki67, pH3 or active Casp-3 expression was automatically detected in cells expressing either H2B-GFP (shSCR tumours) or H2B-RFP (shSOX2 or shNRP1 tumours) using the NIS element software. The percentage of Ki67, pH3 or active Casp-3-positive cells within the lineage was measured in more than 200 fields per condition and plotted in Prism 6. For quantification of division axis, the number of cells analysed ( n ) is indicated in the radial histograms, and included cells from three or more tumours. Axis of division was determined as previously described [49] . Briefly, staining for anaphase/telophase marker Survivin, which localizes to the spindle mid-body, is present at the mid-zone between two daughter nuclei. Angle of division was determined by measuring the angle defined by the plane transecting two daughter nuclei relative to the plane of the basement membrane, as indicated by integrin (CD104/β4 or CD49f/α6 staining) or nidogen staining. Differential gene expression analyses were performed in GenePattern [59] and expression data were visualized in Matlab. Radial histograms of division angle were plotted in Matlab from raw data binned into 10° increments. All other graphs were prepared in Prism 6. Figures were prepared using Adobe Photoshop and Illustrator CS6. Accession codes: Differential gene expression analyses between CSCs, EPI and HFSCs have been deposited at GSE29328 . How to cite this article: Siegle, J. M. et al. SOX2 is a cancer-specific regulator of tumour initiating potential in cutaneous squamous cell carcinoma. Nat. Commun. 5:4511 doi: 10.1038/ncomms5511 (2014).